Imaging and steering an optical wireless nanoantenna link Optical nanoantennas tailor the transmission and reception of optical signals. Owing to their capacity to control the direction and angular distribution of optical radiation over a broad spectral range, nanoantennas are promising components for optical communication in nanocircuits. Here we measure wireless optical power transfer between plasmonic nanoantennas in the far-field and demonstrate changeable signal routing to different nanoscopic receivers via beamsteering. We image the radiation pattern of single-optical nanoantennas using a photoluminescence technique, which allows mapping of the unperturbed intensity distribution around plasmonic structures. We quantify the distance dependence of the power transmission between transmitter and receiver by deterministically positioning nanoscopic fluorescent receivers around the transmitting nanoantenna. By adjusting the wavefront of the optical field incident on the transmitter, we achieve directional control of the transmitted radiation over a broad range of 29°. This enables wireless power transfer from one transmitter to different receivers. Resonant plasmonic metal nanoparticles enable confinement of incident optical fields to the nanoscale and enhancement of radiation from sub-wavelength sources by impedance matching [1] , [2] . In analogy to the radio frequency (RF) domain, such particles are called optical antennas [3] , [4] , [5] . They have led to breakthroughs in enhanced nonlinear frequency conversion [6] , [7] , ultra-sensitive sensing [8] , [9] , [10] , [11] , emission enhancement and radiation engineering of single photons [12] , [13] , [14] , [15] , [16] , [17] , as well as enhanced photo-detection at the nanoscale [18] , [19] . One of the envisioned applications of plasmonics is optical on-chip circuitry [20] , [21] with nanoscale footprints to combine photonics with integrated electronics [22] for high-speed computing and high-bandwidth communication. One approach is the use of plasmonic waveguides. They confine light to a sub-wavelength volume [23] , [24] , [25] , [26] , [27] , [28] , [29] , [30] , [31] , [32] , [33] but suffer from large losses. Moreover, such waveguides realize fixed connections and require complicated multilayer arrangement for high integration density. As an alternative, a wireless link between two nanoantennas as proposed by Alù and Engheta [34] enables large-distance communication because of the absence of absorption losses during propagation. In this work, we present the experimental observation of far-field power transfer via free space between transmitting and receiving optical nanoantennas. We excite the antenna from the far-field ( λ =785 nm) and image the intensity distribution around plasmonic nanoantennas. We demonstrate a significant directivity increase by using antenna arrays instead of single antennas as transmitters. We position nanoscopic fluorescent receivers with nanometer scale accuracy and demonstrate that the attenuation of the transmitted power follows the inverse square power law of radiative beam propagation. With our technique we can measure the signal decay across a range of 20 μm (38 λ in the medium) by mapping the intermediate- and far-field around the transmitter. The measurement range is limited here only by the field of view of the experimental setup. A change of the incident wavefront across the nanoplasmonic antenna array leads to redirection of the intensity over a 29° range, and we demonstrate controllable signal routing to different plasmonic antenna receivers via beamsteering. 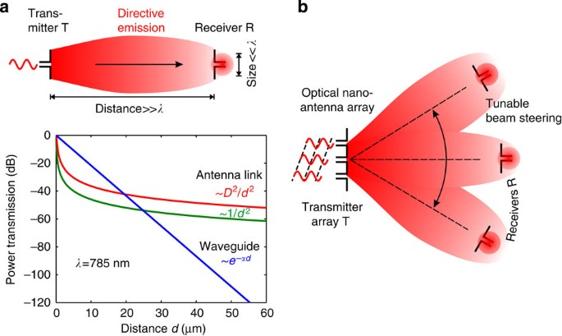Figure 1: Optical antennas for wireless power transfer at the nanoscale. (a) Optical nanoantennas enhance transmission and reception of electromagnetic waves via impedance matching and high directivity, allowing efficient power transfer between source and receiver (top). An optical nanoantenna wireless link exhibits a power-law signal decay (plotted on the bottom, based on ref.34). In comparison, in a plasmonic waveguide the transmitted power decreases exponentially, rendering the signal weaker than in the antenna link for distances larger than approximately 20 μm. Here we consider a case where the attenuation of intensity in the waveguide isα=(2 μm)−1and antenna directivity isD=3. (b) Optical nanoantenna arrays allow beamsteering to address different antenna receivers. Low-loss wireless power transfer with optical antennas Figure 1a depicts the concept of optical power transfer via free-space between transmitting antenna T and receiving antenna R. The lower panel of Fig. 1a compares the power transmission as a function of distance d of such a nanoantenna link (green curve) to a plasmonic waveguide (blue curve). Here we consider an absorption constant α =(2 μm) −1 for lithographically fabricated waveguides with a width of 100 nm at the near-infrared wavelength λ =785 nm (ref. 25 ). There is a trade-off between field confinement and propagation length, for example, for a cylindrical plasmonic waveguide, a decrease in the wire width leads to higher field confinement but results in a strong increase of the losses [35] . In contrast, for the antenna link, absorption losses occur only at the antennas and are thus much lower than for a waveguide. The antenna link performs even better when plasmonic antennas with high directivity D are used as transmitters [15] , [36] and receivers [37] as shown by the red curve in Fig. 1a . In the RF domain, antenna arrays achieve extremely high directivities because of constructive interference of the radiation of the individual antennas. They furthermore enable tuneable redirection, that is, steerability of the transmitted radiation by phasing the individual antennas (see Fig. 1b ) [38] . These properties make antenna arrays irreplaceable in steerable far-distant communication where direct connections are no option. Bringing this concept to the optical frequency domain by employing optical nanoantenna arrays, [39] , [40] opens up a new perspective of realizing low-loss changeable optical interconnects where direct waveguide connections are not suited [3] , [4] , [34] . Figure 1: Optical antennas for wireless power transfer at the nanoscale. ( a ) Optical nanoantennas enhance transmission and reception of electromagnetic waves via impedance matching and high directivity, allowing efficient power transfer between source and receiver (top). An optical nanoantenna wireless link exhibits a power-law signal decay (plotted on the bottom, based on ref. 34 ). In comparison, in a plasmonic waveguide the transmitted power decreases exponentially, rendering the signal weaker than in the antenna link for distances larger than approximately 20 μm. Here we consider a case where the attenuation of intensity in the waveguide is α =(2 μm) −1 and antenna directivity is D =3. ( b ) Optical nanoantenna arrays allow beamsteering to address different antenna receivers. Full size image Imaging and optimizing the radiation pattern We first study and optimize the radiation pattern of the transmitter for our nanoantenna wireless link. The schematic of Fig. 2a shows the geometry of the experiment. We fabricate single gold rod-type nanoantennas and one-dimensional gold nanoantenna arrays on a glass substrate (refractive index n =1.52) by electron beam lithography (see Methods for details). With scanning electron microscopy we determine the length and width of a single antenna element as 100 nm and 50 nm, respectively. Owing to the evaporation process the height of the antenna is 40 nm. The period of the array is 170 nm. We coat the sample with a 60-nm thick layer of PMMA (polymethyl methacrylate) that contains fluorescent molecules ( n =1.48, see Methods for details). Embedding the structure in immersion oil ( n =1.52) eliminates the perturbation of the antenna pattern by the substrate. We can therefore directly measure the antenna radiation in a homogeneous environment via the fluorescence of the dye molecules, which absorb at λ =785 nm (emission maximum around λ =850 nm). The slightly lower refractive index of the PMMA film compared with the surrounding media prevents waveguiding effects. We excite the plasmonic antennas with a tightly focused laser beam ( λ =785 nm) incident along the z axis using an oil immersion objective (numerical aperture=1.4, see Methods for details). The antenna is designed such that at this wavelength, light incident with the polarization set along the long axis of the antenna elements ( x -direction, see Fig. 2a ) leads to excitation of the first order plasmon resonance of the antenna and hence resonant dipolar scattering to the far-field. Setting the polarization along the short axis of the antenna elements ( y -direction) switches the antenna radiation off (see Supplementary Fig. 1 ). 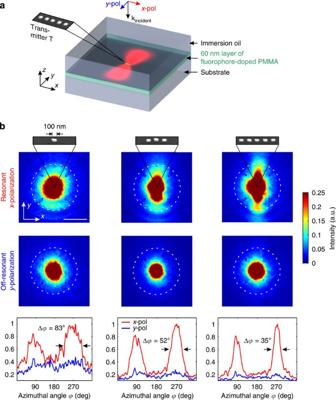Figure 2: Mapping and optimizing the directivity of a single optical nanoantenna array. (a) We map the radiation pattern of a single optical nanoantenna array in a homogeneous medium. The structures are on a glass substrate, which is covered with index matching oil. A 60-nm thick continuous layer of PMMA with fluorescent molecules (IR140) is used to image the radiation pattern in thexy-plane when a tightly focused beam is incident along thezaxis. (b) When the polarization of the incident field is along the long axis of the rod-shaped elements of the antenna array (resonantx-polarization) we observe a directional radiation pattern, which is elongated in they-direction (top row, scale bar 10 μm). In comparison, when the polarization of the incident light is along theyaxis (off-resonanty-polarization) the fluorescence pattern is circular stemming from the direct excitation of the molecules by the incident beam (middle row). As the number of antenna elements is increased the antenna radiation pattern narrows significantly due to higher directivity as seen in the plot of the fluorescence intensity along the white dashed circles (bottom row). Figure 2: Mapping and optimizing the directivity of a single optical nanoantenna array. ( a ) We map the radiation pattern of a single optical nanoantenna array in a homogeneous medium. The structures are on a glass substrate, which is covered with index matching oil. A 60-nm thick continuous layer of PMMA with fluorescent molecules (IR140) is used to image the radiation pattern in the xy -plane when a tightly focused beam is incident along the z axis. ( b ) When the polarization of the incident field is along the long axis of the rod-shaped elements of the antenna array (resonant x -polarization) we observe a directional radiation pattern, which is elongated in the y -direction (top row, scale bar 10 μm). In comparison, when the polarization of the incident light is along the y axis (off-resonant y -polarization) the fluorescence pattern is circular stemming from the direct excitation of the molecules by the incident beam (middle row). As the number of antenna elements is increased the antenna radiation pattern narrows significantly due to higher directivity as seen in the plot of the fluorescence intensity along the white dashed circles (bottom row). Full size image We record wide-field images of the luminescence to observe the antenna radiation pattern [41] . The top row of Fig. 2b displays the luminescence pattern around a single dipole transmitter (left), a three dipole array transmitter (centre), and a five dipole array transmitter (right). The transmitter is located in the centre of each 30 × 30 μm 2 wide-field image. The fluorescence pattern is elongated along the y -direction for all three transmitters when the polarization of incident light is along the x axis (resonant polarization). The pattern becomes more elongated with increasing number of elements in the array as the directivity of the transmitting array increases. In the middle row, we show as reference the fluorescence pattern for incident y -polarized light (off-resonant polarization), which is circular for all transmitters. Here, the polarization is along the short-axes of the nanorods and the off-resonant antenna radiation is too weak to be detected in this case. The measured luminescence stems from direct excitation of the dye molecules by the incident laser beam. We find that the fluorescence signal does not scale linearly as a function of the power of the incident light because of bleaching and saturation. We take both effects into account in our theoretical model (see Methods for a discussion of this and details about the model). In Supplementary Fig. 2, we compare measured and calculated antenna patterns for transmitter arrays with different number of antenna elements. The experimental data agree very well with the theoretical patterns. In the bottom row of Fig. 2b we plot the fluorescence intensity along a circular path 9 μm away from the transmitter. We observe two maxima at the azimuthal angles 90° and 270° ( y axis) for the resonant polarization (red curves), which are not present for off-resonant polarization (blue curves). From these data, we extract the angular width Δ φ of the luminescence pattern, which we define as the full width at half maximum of the peak at 270° excluding the offset because of direct excitation of the molecules by the incident laser beam. It decreases for resonant polarization from 83° for the single dipole antenna to 35° for the five dipole array demonstrating increased directivity for the antenna array in close analogy to what is achieved in RF engineering [38] . The dipolar patterns of each antenna element add up constructively in the 90° and 270° directions, resulting in the narrowing of the scattered intensity. We have also investigated nanoantenna arrays with two and four dipoles (see Supplementary Fig. 2 ). We conclude that the reduction of Δ φ saturates in our geometry for five elements in the array (see Supplementary Fig. 2 ). The reason for this is that for larger arrays the outermost antennas are not efficiently excited by the incident tightly focused laser beam and do not contribute to the radiation pattern. We extract the directivity [3] from our calculated pattern (for details on the model see Supplementary Fig. 2 and Methods ) and find a maximum of 3.6 along the y -direction for the five-dipole array. Here we use as basic element a simple dipole antenna. In the future, more sophisticated designs of transmitting [15] , [36] and receiving antennas [37] as well as array configurations, for example, two-dimensional arrays [39] , [40] , will boost the directivity and thus power transfer between transmitter and receiver even further. Studying the radiation pattern of such sophisticated optical antenna configurations can be achieved by using our presented fluorescence method. Optical antennas for nanoscale wireless power transfer We now use the five-dipole nanoantenna array in a nanophotonic wireless link to study power transfer between a nanoantenna transmitter and receiver. We fabricate sub-wavelength-sized luminescent receivers at different distances to the transmitter as shown in Fig. 3a . This is achieved by blending fluorescent molecules into electron-beam resist and then patterning disks with nominally 250 nm diameter and 60 nm height (see Methods). We use a two-step electron-beam process to position the receivers with 10 nm accuracy in a chain along the transmission direction of the transmitter. The structure is again covered with immersion oil so that the transmitted radiation is not deflected into the substrate. We excite the transmitter and record wide-field luminescence images to observe power transfer to the receivers. A schematic of the configuration is depicted in Fig. 3b together with a luminescence image of the sample when we excite the transmitter. In Fig. 3c , we show the luminescence intensity as a function of distance d from the transmitter (blue circles). Comparison of our experimental data to a 1/ d 2 decay (green line, see also Fig. 1a ) confirms that we observe power transfer via radiative propagation. To enlarge the dynamic range of our measurement, we record luminescence images with increasing power of the excitation. For low-excitation power, the luminescence of the receivers close to the transmitter scales linearly with the excitation power and the dye is not significantly bleached. As the excitation power is increased, this linear regime is shifted to larger distances from the transmitter, allowing us recording data with high signal-to-noise ratio over the whole distance range. We normalize the luminescence signal with the respective excitation power value and plot the data in Fig. 3c (see Methods for further details). The used excitation power is encoded in the brightness of the data points. To realize a plasmonic nanoantenna link, we now use our method to position a fluorescent disk on top of a gold nanodisk as receiving antenna. The receiving antenna is designed to be resonant at λ =785 nm (that is, 130 nm diameter and 40 nm height). The fluorescence image in Fig. 3b shows that at a distance of 20 μm away from the transmitter, at the location of the plasmonic receiver antenna, we observe a distinct signal increase with the luminescence intensity being comparable to the signal from the receivers positioned at 6 and 8 μm distances. This corresponds to a 7.5 × receiving signal enhancement (circles with red rim in Fig. 3c ) when compared with a fluorescent disk without receiving antenna. We remark that this underestimates the enhancement. The nominal size of the fluorescent disks is the same for the receivers with and without a plasmonic antenna. Thus, the number of fluorescent molecules is smaller for the receiver with a plasmonic antenna, which occupies part of the volume of the fluorescent receiver. The signal enhancement depends on the overlap of the sub-wavelength receiver dye disk and the hotspot of the plasmonic antenna and can be tailored by antenna design, the size of the dye receiver and its respective position to the antenna. To estimate the efficiency of the link, we compare the signal at the receiving antenna with the signal that we obtain when exciting a dye disk directly with the incident laser. We find a total power transfer efficiency of 10 −4 . This estimation includes the scattering efficiency of our transmitter and how efficiently we can drive it from the far-field. The wireless signal transmission itself between transmitter and receiver is therefore more efficient. It is furthermore straightforward with our technique to employ more sophisticated antenna designs in an optical nanoantenna link and image the signal transfer. Our method can be extended to couple few or even single quantum emitters with great positioning accuracy to transmitting nanoantennas [15] , realizing on-chip wireless and nanoscale single photon transmission and reception. 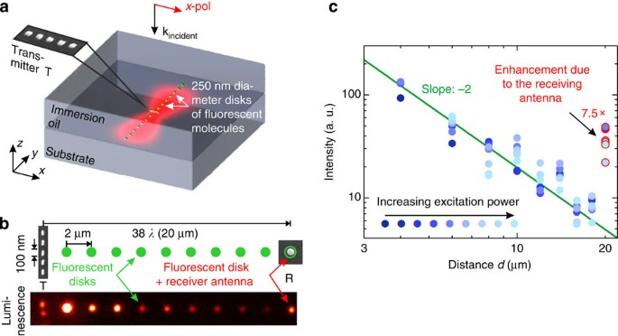Figure 3: Wireless power transfer using optical nanoantennas. (a) We fabricate localized receivers that consist of 250 nm diameter and 60 nm high luminescent disks along the direction of the beam transmitted from a five-element optical antenna array. The transmitter is excited by a tightly focused beam polarized along the resonantx-direction of the antenna array resulting in radiation directed along theyaxis. (b) In the fluorescence image of the structure, we observe a decay of emission from the receivers as a function of distance from the transmitter except for the distance of 38 λ where the receiver is equipped with a plasmonic receiving antenna. (c) The emission intensity normalized to the excitation power decreases linearly as a function of distance from the transmitter in a double logarithmic plot. The experimental data are in good agreement with the 1/d2power-law model for free-space links (green curve). For the antenna-to-antenna link, we observe a factor of 7.5 signal enhancement because of the receiving plasmonic antenna (circles with red rim). To increase the dynamic range of the experiment, we record luminescence images at increasing excitation power (see Methods for details on data analysis). Figure 3: Wireless power transfer using optical nanoantennas. ( a ) We fabricate localized receivers that consist of 250 nm diameter and 60 nm high luminescent disks along the direction of the beam transmitted from a five-element optical antenna array. The transmitter is excited by a tightly focused beam polarized along the resonant x -direction of the antenna array resulting in radiation directed along the y axis. ( b ) In the fluorescence image of the structure, we observe a decay of emission from the receivers as a function of distance from the transmitter except for the distance of 38 λ where the receiver is equipped with a plasmonic receiving antenna. ( c ) The emission intensity normalized to the excitation power decreases linearly as a function of distance from the transmitter in a double logarithmic plot. The experimental data are in good agreement with the 1/ d 2 power-law model for free-space links (green curve). For the antenna-to-antenna link, we observe a factor of 7.5 signal enhancement because of the receiving plasmonic antenna (circles with red rim). To increase the dynamic range of the experiment, we record luminescence images at increasing excitation power (see Methods for details on data analysis). Full size image Steering the optical nanoantenna link We now illustrate the key advantage of wireless power transfer over fixed nanoscale connections by demonstrating the rerouting of optical signals across large distances to different nanoscopic receiving points via beamsteering. This requires controlling the shape of the incident wavefront on the nanoscale. The tightly focused incident light exhibits a steep curvature of the incident wavefronts close to the focal plane. This results in a phase difference between neighbouring array elements as shown in the top row of Fig. 4a . By moving the focus away from the sample plane (Δ z =−1 μm) and shifting the lateral position of the incident beam with respect to our antenna array, we introduce a controlled phase gradient across the nanoantenna array [42] . The bottom row of Fig. 4a shows the phase distribution in the xy -plane for Δ z =−1 μm. We fabricate a transmitter array in the centre of a 20-μm diameter ring of 250 nm diameter fluorescent receiver disks. Every second receiver contains a plasmonic nanodisk antenna (see Supplementary Fig. 3 ) that acts as resonant receiver. In Fig. 4b we display the luminescence images of the link for different values of the incident beam shift s . When the incident beam is positioned at s =0 nm, the transmitted beam is directed along the y direction and the receivers in this direction light up (centre). The receivers with plasmonic antennas luminesce up to six times more intensely when compared with receivers without plasmonic antennas. Shifting the beam to s =−400 nm ( s =+400 nm) steers the transmitted beam towards the left (right) receiving antennas (see also Supplementary Fig. 4 ). 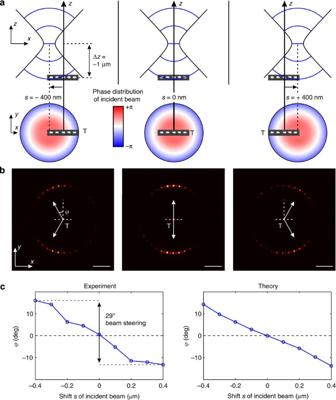Figure 4: Beamsteering to address different antenna receivers. (a) The phase of the elements of the transmitter nanoantenna array is adjusted by displacing the focus of the incident tightly focused beam from the centre of the antenna array. When the microscope objective is slightly defocused, the wavefronts of the incident light field are curved (blue wavefronts in the top schematic correspond toλspacing). Displacing the focused beam laterally leads to a phase gradient across the antenna. The scanning electron micrographs of the antenna array T are to scale with the calculated wavefronts and phase distributions. (b) As a result of the beamsteering different antenna receivers light up depending on the beam direction, which is observed in luminescence images of a 10-μm ring of luminescent receivers around the transmitter array (scale bar 5 μm). Every second receiver is equipped with a receiving plasmonic antenna, leading to an enhancement of the signal by a factor of 6 (see alsoSupplementary Fig. 3). (c) We obtain a total beamsteering range of 29° as determined from measurements on a continuous luminescent film (seeSupplementary Fig. 5andSupplementary Movie 1). The experimental results are in good agreement with the theoretical prediction obtained by using the model for the luminescence signal (see Methods). Figure 4: Beamsteering to address different antenna receivers. ( a ) The phase of the elements of the transmitter nanoantenna array is adjusted by displacing the focus of the incident tightly focused beam from the centre of the antenna array. When the microscope objective is slightly defocused, the wavefronts of the incident light field are curved (blue wavefronts in the top schematic correspond to λ spacing). Displacing the focused beam laterally leads to a phase gradient across the antenna. The scanning electron micrographs of the antenna array T are to scale with the calculated wavefronts and phase distributions. ( b ) As a result of the beamsteering different antenna receivers light up depending on the beam direction, which is observed in luminescence images of a 10-μm ring of luminescent receivers around the transmitter array (scale bar 5 μm). Every second receiver is equipped with a receiving plasmonic antenna, leading to an enhancement of the signal by a factor of 6 (see also Supplementary Fig. 3 ). ( c ) We obtain a total beamsteering range of 29° as determined from measurements on a continuous luminescent film (see Supplementary Fig. 5 and Supplementary Movie 1 ). The experimental results are in good agreement with the theoretical prediction obtained by using the model for the luminescence signal (see Methods). Full size image We achieve continuous beamsteering of the transmitted radiation as shown in the left panel of Fig. 4c where we plot the transmitted beam-direction φ in the xy -plane as a function of incident beam shift s . The beamsteering angle φ is extracted from wide-field fluorescence images similar to the ones of Fig. 2b where we visualize the full radiation pattern in the xy -plane (see Supplementary Fig. 5 and Supplementary Movie 1 for the images). We find a 29° beamsteering range, which is in very good agreement with theory. We note that the shaping of the incident wavefront in our experiment can be made actively, for example, with a liquid crystal modulator, enabling dynamic and fast switching signal distribution. To achieve coherent feeding of our antenna array from nanoscopic sources instead from the far-field, we envision coupling of nonlinear frequency conversion nanoparticles, which can be driven in-phase with the illuminating laser spot, to the individual antenna elements [43] . Beamsteering and directive radiation as demonstrated would then work in concert with nanoscopic excitation of our antennas. Another approach is the implementation of our wireless signal transfer scheme in a nanoscopic photonic circuit using plasmonic waveguides as feeding lines [21] , [44] , where the phase can be actively [45] adjusted. This combines low-loss antenna links for reconfigurable long-distance signal transmission with integrated plasmonics for nanoscale routing of light. We have applied the powerful concepts in RF engineering of high directivity wireless signal transfer and beamsteering to the optical wavelength regime. In the quest for reconciling the size mismatch between diffraction-limited integrated photonics and integrated electronics, our results on wireless power transfer in tunable optical nanoantenna links prelude long-distance and flexible optical communication at the nanoscale. By modulating the amplitude of the input signal, high-speed information transfer can be easily achieved in our experiment because of the very short response time of the dye molecules (on the order of nanoseconds). The nanoscopic footprint of our nanoantenna array allows for high integration densities of optical interconnects without suffering from electromagnetic interference. Multilayer geometries can be avoided, implying that inter- and intra-chip communication can be designed more efficiently by multiple links with crossing paths on the same layer. Plasmonic nanoantennas are broadband, allowing for wavelength multiplexing to increase the data transfer rate. In addition, control over polarization could add another degree of freedom and would increase the possibilities to encode transmitted data even further. The presented approach using fluorescent dye molecules patterned with electron-beam lithography is immediately applicable to image and to quantitatively analyse signal transfer to nanoscopic receivers in various geometries [46] , [47] and can be applied to couple different quantum systems across large distances via optical antennas, for example, in a donor–acceptor configuration [48] , [49] . Sample fabrication Plasmonic antenna samples are prepared with electron beam lithography on a microscope cover glass. We spin coat first a 200-nm thick double layer PMMA (chain lengths 250,000 and 950,000) and then a 30-nm thick layer of conductive polymer (eSpacer 300Z) to avoid charging of the sample during exposure. After exposure and development, 2 nm chromium as adhesion layer and 40 nm of gold are thermally evaporated. A lift-off process removes the excess metal. For the fluorescent film, IR140 (Sigma-Aldrich) is blended into PMMA (950,000 chain length) at a concentration of 2 mg ml −1 and spin coated on the sample, forming a 60-nm thick layer. For the fluorescent disks, IR140 is blended into ARN 7520 resist (Allresist) at a concentration of 2 mg ml −1 . We then use alignment marks, which we have processed together with the gold antennas in order to align the coordinate system in a second electron beam lithography step. This allows us to pattern 60 nm high-fluorescent disks and to position them with 10 nm accuracy [50] . As a final step, we cover the sample with immersion oil (Olympus). Sample characterization Experiments were performed with a home-built fluorescence microscope. We use 785 nm laser diodes (Spindler & Hoyer and Roithner Lasertechnik) as excitation sources. The single-mode laser beam is expanded so that it completely fills the aperture of our objective. We use a Nikon CFI Plan Apo VC × 100 oil immersion objective with a numerical aperture of 1.4 to focus onto the sample. From measurements on gold nanoparticles we determine the full-width half-maximum of the spot in the focus to 300 nm. A polarizer and a removable λ /2 plate control the incident polarization, and a mirror mounted on a galvanometer is used to adjust the position of incident beam with respect to the antennas. Luminescence light is collected by the same objective and filtered from the excitation light with a dichroic beam-splitter (Semrock) and long-pass filter (Chroma). Wide-field images of the sample plane are taken with a nitrogen-cooled CCD camera (Roper Scientific). Modelling the antenna pattern reported via the luminescence signal For resonant polarization ( x -polarization), the field that excites the molecules around the transmitter array consists of the incident beam and the field radiated by the antenna. For off-resonant polarization ( y -polarization), the contribution from the antenna is absent. The incident field is calculated using the vectorial complex field description of a focused Gaussian laser beam [51] . We describe the scattered field from our antenna array using the discrete-dipole approximation [52] , where each antenna element is considered as a single dipole. We take the polarizability of the dipoles from numerical simulations [53] . The induced dipole moments of the antenna elements are calculated self-consistently, taking into account the coupling between the dipoles. The field radiated by the antenna array is the sum of the complex fields of all dipole elements. For the beamsteering, we take into account the shift of the incident driving field, which leads to a phase gradient across the array (see Fig. 4 and Supplementary Fig.5 ). Finally, the total intensity I ( r ) around the transmitter is then proportional to the squared absolute of the sum of the complex incident field and the sum of the complex fields of all dipole elements where we introduce the parameter a to weigh the relative strength of the incident field with respect to the field radiated by the antenna. In this way, we take into account differences between the realized structures and the ideal antennas for which the polarizability was calculated numerically. The measured luminescence signal s ( t , r ) does not scale linearly with the intensity I ( r ) around the transmitter because of saturation and bleaching of the dye molecules. We take this into account using the nonlinear equation Here, s ( t 0 , r ) is the signal obtained by collecting the emission for a duration Δ t starting at time t 0 . Saturation of the signal is taken into account in the term , where I s is the saturation intensity. We assume a double exponential decay due to bleaching. The starting concentration of molecules bleaching with intensity-dependent decay rates c 1 f ( I ( r )) and c 2 f ( I ( r )) are denoted s 1 and s 2 , respectively. Fitting the antenna pattern We use Equation (2) to fit our experimental luminescence images to the model. To obtain the parameters characterizing the luminescent molecules, I s , s 1 , s 2 , c 1 and c 2 , we fit the experimental data for the five-dipole antenna array to the theory. The data and result of the fit are shown in the right most column of Supplementary Fig. 2a . We then use these parameters to fit all the other data to the model using a as the only fitting parameter. This accounts for small variations in the fabricated devices. For the beamsteering pattern shown in Supplementary Fig. 5, we again use the parameters obtained from the five-dipole array fit. The incident field exciting the transmitter is calculated using the rigorous theory of focusing of vectorial beams as described above taking into account the shift of the focal spot away from the centre of the nanoantenna array. The parameter a is again the only parameter used in the fitting. For all the intermediate beam shifts between s =−400 nm and s =+400 nm, we calculate the patterns with the fitted parameters and extract from the pattern cross sections (see Fig. 2 ) the beam direction in which the maximum intensity occurs to obtain the theory plot in Fig. 4c . Data analysis and visualization For the experimental luminescence images of the continuous films ( Fig. 2b , Supplementary Fig. 2 and Supplementary Fig. 3 ), we plot the raw data from which the background was subtracted. The background was acquired with the laser turned off during image acquisition. The images are normalized to the maximal value of the luminescence for x -polarized excitation. We recorded ten images with an integration time of 10 s for each image and alternating polarization ( x -pol and y -pol) of the incident beam. The cross-sections in Fig. 2b and Supplementary Fig. 2 were obtained by first interpolating the raw data on a ring with radius r around the transmitter antenna. The interpolated data were then averaged for different rings with r ranging from 8.5 to 9.5 μm to obtain the values that are plotted in Fig. 2b and Supplementary Fig. 2 . Analysis of the beam width at different r leads to similar results. In the experiment of Fig. 3 we used excitation powers 1, 5, 10, 20, 30, 40, 50, 60, 70 and 80 μW. In Fig. 3b we plot the raw data for the highest excitation power with background subtraction as described above. For Fig. 3c we first determine the signal for each receiver by summing up the luminescence signal in the pixels falling within a 700-nm diameter area around each receiver. We obtain the background signal for each receiver by taking mean signal on a circular disk around the receiver with inner diameter of 1,000 nm and outer diameter of 1,400 nm. We estimate the noise of our images from the standard deviation of the background signal. We plot the signal for the receivers where the ratio of the signal per pixel to noise is above 2. We measure the contribution from direct excitation of the receiver by the incident laser beam using receivers placed in the orthogonal ( x -) direction. We compare for each distance the signal for receivers in the x - and y -directions and exclude the data points for which the ratio of the two is larger than 0.3. To obtain the green line in Fig. 3c we take the mean of the signals at each distance and fit the offset y 0 of a y 0 / d 2 decay. The enhancement owing to receiving antenna is calculated by taking the ratio of the mean of the antenna signals and the intensity of the green line at 20 μm. We assume that the infrared emission because of gold luminescence of the receiving antenna is negligible in our experiment because the incident power on the receiving antenna is rather low [54] . The measured enhancement factor in luminescence is therefore solely due to the field confinement. For the highest excitation power of 80 μW, we determine the maximal distance where we can still observe signal transfer to 162 μm without receiving antenna and 443 μm with receiving antenna. At these distances, the extrapolated signal becomes equal to the noise. Here the noise was taken for the receiver at a distance of 20 μm. To observe signal transfer even further away, the excitation power can be increased. The luminescence images shown in Fig. 4b were obtained by subtracting the wide-field images for resonant x - and non-resonant y -polarization to eliminate the contribution of direct excitation via the incident laser beam. How to cite this article : Dregely, D. et al. Imaging and steering an optical wireless nanoantenna link. Nat. Commun. 5:4354 doi: 10.1038/ncomms5354 (2014).